Nitrate formation from atmospheric nitrogen and oxygen photocatalysed by nano-sized titanium dioxide The concentration of nitrate in aquatic systems is rising with the development of modern industry and agriculture, causing a cascade of environmental problems. Here we describe a previously unreported nitrate formation process. Both indoor and outdoor experiments are conducted to demonstrate that nitrate may be formed from abundant atmospheric nitrogen and oxygen on nano-sized titanium dioxide surfaces under UV or sunlight irradiation. We suggest that nitric oxide is an intermediate product in this process, and elucidate its formation mechanisms using first-principles density functional theory calculations. Given the expanding use of titanium dioxide worldwide, such a titanium dioxide-mediated photocatalysis process may reveal a potentially underestimated source of nitrate in the environment, which on one hand may lead to an increasing environmental pollution concern, and on the other hand may provide an alternative, gentle and cost-effective method for nitrate production. Our understanding of the nitrogen cycle has shifted from how to enhance nitrogen fixation to promote the production of food and energy to the realization that an elevated level of reactive nitrogen poses a growing influence on human health and environmental systems [1] , [2] . Human activities such as fossil fuel combustion, industrial nitrate production, the use of artificial nitrogen fertilizers and the release of nitrogen in waste have drastically altered the global nitrogen cycle [1] , [3] . The Haber–Bosch and Ostwald processes are the most well-known industrial nitrate-producing methods for making fertilizer from nitrogen (N 2 ) in the presence of noble metal catalysts at high temperatures and pressures [4] , [5] . However, an excess level of nitrate emitted into drinking water systems is toxic to humans, for example, resulting in ‘blue baby syndrome’ in children [6] . It can also lead to eutrophication and algae blooms in freshwater and estuaries [1] , [2] , [6] . Nano-sized titanium dioxide (TiO 2 <100 nm) is used as an additive worldwide because of its high refractive index, strong UV-light-absorbing capability, and superior sterilizing, deodorizing and anti-fouling properties [7] , [8] . It accounts for 70% of the total production of pigments worldwide. Millions of tons of TiO 2 are produced annually and its production is expected to increase continually [9] , [10] . TiO 2 nanomaterials, widely used in white paints, foods, consumer products and household products, are disposed of down drains, discharged in faeces/urine, washed off of surfaces, discharged into sewage and eventually enter wastewater-treatment plants. Furthermore, the intake of nanoscale TiO 2 through foods by human beings is estimated to be on the order of 1 mg Ti per kg of body weight per day, with children identified as having a higher exposure rate because of the greater content of nanoscale TiO 2 in sweets [10] . Thus far, TiO 2 has been widely used as an environmentally friendly photocatalyst and additive [10] , [11] , [12] , [13] . However, there has been no report on direct nitrate production from atmospheric N 2 and O 2 through TiO 2 -mediated photocatalysis under ambient conditions and its potential negative influence on the environment, given its increasing use worldwide. In this study, we conduct both indoor and outdoor experiments to explore potential environmental pollution problems induced by such a TiO 2 -mediated photocatalysis, and to establish a cost-effective photocatalytic process for nitrate production. The first-principles density functional theory calculations are applied to elucidate the formation mechanisms of intermediate gas products on the (001) surface of nano-TiO 2 . The results suggest that nano-sized titanium dioxide may catalyse the formation of nitrate via the photochemical reaction of atmospheric nitrogen and oxygen. Photocatalytic nitrate production Scanning electron microscopy was used to image the surface morphology and structure of the TiO 2 -carbon paper used in the photocatalytic process. The carbon paper covered with TiO 2 displayed a cracked-mud structure, resulting in an increased actual surface area ( Fig. 1a,b ). The X-ray diffraction spectrum of the TiO 2 , in which the peaks correspond to anatase and rutile phases ( Fig. 1a,b ), exhibited the same structure as that of the commercial TiO 2 nanoparticles. P25 is a 15/85 mixture of rutile/anatase, whereas E171 is anatase. This result indicates that the coating of TiO 2 on the carbon paper surface did not change the structure of the TiO 2 . 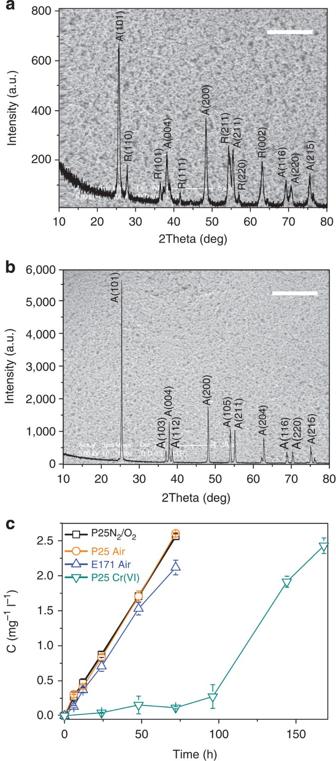Figure 1: Structural characterization of TiO2and nitrate concentration profiles. (a) Scanning electron microscopy image and X-ray diffraction spectrum of the P25 on the TiO2-carbon paper, scale bar, 5 μm; (b) scanning electron microscopy image and X-ray diffraction spectrum of the E171 on the TiO2-carbon paper; A represents anatase and R represents rutile, scale bar, 10 μm; and (c) concentration profiles of nitrate in the open photocatalytic reactor filled with ultrapure water (P25 N2/O2: the N2/O2(3:1/v:v) mixture was purged into the reactor with the P25-carbon paper inserted; the tests were conducted in triplicate; the error bar at each data point reflects the s.d. of the three repeated measurement of concentrations. P25 Air: air was purged into the reactor with the P25-carbon paper inserted; E171 Air: air was purged into the reactor with the E171-carbon paper inserted; P25 Cr(VI): air was purged into the reactor with the P25-carbon paper inserted and 0.01 mM Cr2O72−was dosed as an electron scavenger). Figure 1: Structural characterization of TiO 2 and nitrate concentration profiles. ( a ) Scanning electron microscopy image and X-ray diffraction spectrum of the P25 on the TiO 2 -carbon paper, scale bar, 5 μm; ( b ) scanning electron microscopy image and X-ray diffraction spectrum of the E171 on the TiO 2 -carbon paper; A represents anatase and R represents rutile, scale bar, 10 μm; and ( c ) concentration profiles of nitrate in the open photocatalytic reactor filled with ultrapure water (P25 N 2 /O 2 : the N 2 /O 2 (3:1/v:v) mixture was purged into the reactor with the P25-carbon paper inserted; the tests were conducted in triplicate; the error bar at each data point reflects the s.d. of the three repeated measurement of concentrations. P25 Air: air was purged into the reactor with the P25-carbon paper inserted; E171 Air: air was purged into the reactor with the E171-carbon paper inserted; P25 Cr(VI): air was purged into the reactor with the P25-carbon paper inserted and 0.01 mM Cr 2 O 7 2− was dosed as an electron scavenger). Full size image In the photoreactor under UV irradiation, the nitrate concentration increased almost linearly with the reaction time when purified air or N 2 /O 2 (3:1/v:v) gas was purged into the reactor, and an average nitrate-producing rate of 3.51±0.06 mg m −2 h −1 was obtained in the two cases using the P25-carbon paper ( Fig. 1c ). The tests with N 2 /O 2 gas confirmed that nitrate was directly formed from N 2 and O 2 through the TiO 2 -mediated photocatalysis. In addition, the similar levels of the nitrate-producing rate in both systems indicate that the interference of nitrogen oxides in the purified air was negligible for all the indoor experiments. For the E171-carbon paper, the rate decreased to 2.96±0.11 mg m −2 h −1 . With the dose of Cr(VI) as an electron scavenger [14] , the rate decreased to 0.29±0.08 mg m −2 h −1 in the initial 96 h, but then increased to 3.42±0.63 mg m −2 h −1 after Cr(VI) became exhausted ( Fig. 1c ), implying that the photogenerated electrons (e − ) might have an important role in such a nitrate-producing process. No nitrate was detected in the reactor when purified air or ultrapure N 2 gas was injected but without photocatalysis (that is, in the absence of UV irradiation, in the presence of UV and carbon paper but without TiO 2 , or without carbon paper and TiO 2 at all). In addition, no nitrate was formed when ultrapure Ar gas was injected and UV irradiation carried out. However, a small amount of nitrate with an average producing rate of 0.18±0.06 mg m −2 h −1 was detected when ultrapure N 2 gas was injected in the presence of UV irradiation. No detectable ammonia or nitrite was measured in all the experiments. These results indicate that the photocatalytic nitrate-producing reaction occurred with the catalysis by P25 or E171 under UV irradiation. Thus, purified air was directly used in the subsequent indoor experiments. The nitrate-producing rate decreased slightly over time, which was attributed to the acidification of the photocatalyst surface. Photocatalytic nitrate production under ambient conditions In the well-controlled climatic chamber at fixed illumination intensity, the nitrate-producing rate initially increased with the increasing relative humidity but decreased once the relative humidity reached a certain height ( Fig. 2a ). Nitrate production also occurred under solar illumination due to the presence of UV light in sunshine ( Fig. 2b,c ). Furthermore, the nitrate-producing rate was closely correlated with the sun illumination intensity at a constant relative humidity (100%), which was achieved through sprinkling ultrapure water on the TiO 2 -carbon paper surface. More nitrate was harvested at noontime (11:00–13:30) and afternoon (13:30–16:00) when a higher illumination intensity was available, compared with that in the morning (8:30–11:00) and at evenfall (16:00–18:30) ( Fig. 2b ). 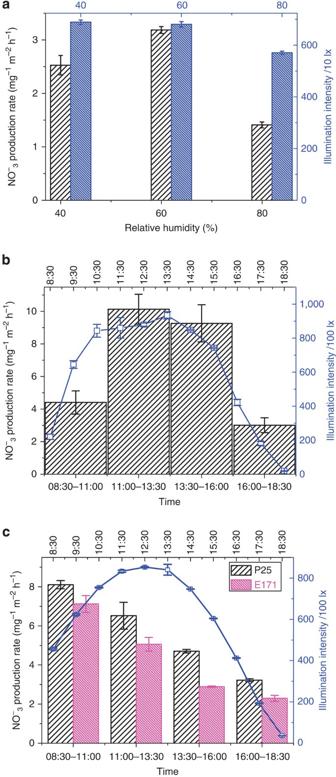Figure 2: Profiles of nitrate production rate under various conditions. (a) Effects of relative humidity on the nitrate production rate and illumination intensity in the climatic chamber; (b) profiles of nitrate production rate and illumination intensity of sunlight in the outdoor photocatalytic process under sunlight irradiation with ultrapure water dropped upon the TiO2(P25)-carbon paper surface on 20 September 2010, in Hefei, China (31.51 °N, 117.17 °E) and (c) profiles of nitrate production rate and illumination intensity of sunlight in the outdoor photocatalytic process under sunlight irradiation without the dropping of ultrapure water on the TiO2-carbon paper surface on 26 July 2012, in Hefei, China. All the tests were conducted in triplicate, and the error bars indicate the s.d. of three repeated measurements. Figure 2: Profiles of nitrate production rate under various conditions. ( a ) Effects of relative humidity on the nitrate production rate and illumination intensity in the climatic chamber; ( b ) profiles of nitrate production rate and illumination intensity of sunlight in the outdoor photocatalytic process under sunlight irradiation with ultrapure water dropped upon the TiO 2 (P25)-carbon paper surface on 20 September 2010, in Hefei, China (31.51 °N, 117.17 °E) and ( c ) profiles of nitrate production rate and illumination intensity of sunlight in the outdoor photocatalytic process under sunlight irradiation without the dropping of ultrapure water on the TiO 2 -carbon paper surface on 26 July 2012, in Hefei, China. All the tests were conducted in triplicate, and the error bars indicate the s.d. of three repeated measurements. Full size image The photocatalytic reaction under ambient conditions was affected by the relative humidity and the sun illumination intensity. The greatest nitrate-producing rate was obtained in the morning (8:30–11:00) with the highest relative humidity and medium illumination intensity. The rate decreased with the reduced illumination intensity from noontime (11:00–13:30) to evenfall (16:00–18:30), which had almost the same relative humidity levels ( Fig. 2c and Supplementary Fig. S2a ). These results imply that such a nitrate-producing process could occur on the surface of ubiquitous areas coated with TiO 2 under ambient conditions, and that the reaction rate is closely associated with the relative humidity and sun illumination intensity. Detected intermediate products A continuous nitrate-producing reaction was also observed in the photocatalytic experiments carried out in the airtight glass reactor with a quartz glass window ( Fig. 3a ). Compared with the chromatogram of the gas in the 5-l flask before and after the photocatalytic reaction, an intermediate gaseous product was detected with a retention time of 1.25 min, which was identified as NO by the Fourier transform IR (FTIR) analysis ( Fig. 3b ). The FTIR analysis of the gas post reaction revealed an increase in the NO concentration of 200 ppb, compared with the samples analysed before the reaction (see Supplementary Fig. S2b, c ). No N 2 O was detected during this process. Thus, NO was the detected intermediate product in this photocatalytic process. 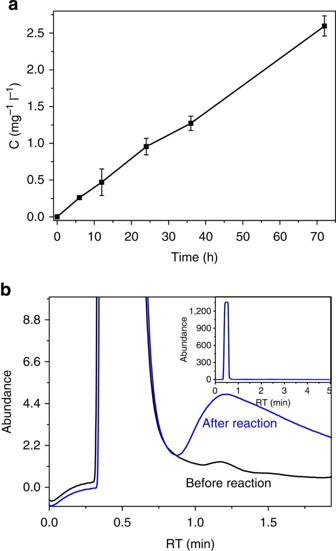Figure 3: Concentration of nitrate and gas chromatogram. (a) Concentration profiles of nitrate in the airtight glass reactor; the tests were conducted in triplicate and (b) partial enlargement chromatogram of the gas in the airtight reactor before and after the reaction with its entire range shown in the inset. The error bars inarefers to the s.d. of three measurements of nitrate concentrations. Figure 3: Concentration of nitrate and gas chromatogram. ( a ) Concentration profiles of nitrate in the airtight glass reactor; the tests were conducted in triplicate and ( b ) partial enlargement chromatogram of the gas in the airtight reactor before and after the reaction with its entire range shown in the inset. The error bars in a refers to the s.d. of three measurements of nitrate concentrations. Full size image Theoretical analysis of photocatalytic mechanisms The above observations suggest that NO was the initial product of this type of photocatalytic process on a TiO 2 surface. The reaction in the presence of Cr(VI) indicates that photogenerated electrons (e – ) had an important role in this process, although the involvement of photogenerated holes (h + ) could not be neglected. Thus, the following photocatalytic NO formation is proposed. The intermediate formation pathways (1) and (2) illustrated in Supplementary Fig. S1 show the reactions occurring with O 2 and e – on the conduction band (CB), and with H 2 O and h + on the valence band (VB) of the TiO 2 (001) surface ( Supplementary Fig. S3 ), respectively. To explore the mechanism that has plausible energies and barriers, a number of mechanistic scenarios have been examined. We first describe the results concerning the preferred reaction mechanism on the CB ( Supplementary Fig. S1 ). The geometry structures of the optimized key reaction intermediates are illustrated in Supplementary Fig. S4 (1~5) for each step of NO formation (detailed description is given in Supplementary Note 1 ). In the photocatalytic process, the Δ r G m θ values of the elementary step and overall process ( Supplementary Table S1 ) indicate that the NO formation on the CB of the TiO 2 (001) surface is thermodynamically favourable compared with the positive Δ r G m θ (173.38 kJ mol −1 ) without added photolytic energy. Moreover, Δ r G m becomes more negative with the increasing temperature ( Supplementary Fig. S5 ), indicating that a high temperature is beneficial to this process. The lower energy barrier ( E a ) of the photocatalytic NO formation reaction shown in the overall potential energy graph ( Fig. 4a ) reveals that the pathway of the CB mechanism is an energetically feasible reaction with a higher reaction rate. 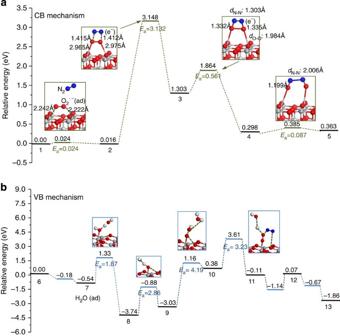Figure 4: Calculated potential energy profile for NO formation. Calculated potential energy profile of each step for NO formation on the conduction band (a) and the valence band (b) of TiO2(001) surface, according toSupplementary Fig. S1. Figure 4: Calculated potential energy profile for NO formation. Calculated potential energy profile of each step for NO formation on the conduction band ( a ) and the valence band ( b ) of TiO 2 (001) surface, according to Supplementary Fig. S1 . Full size image As described in the preferred VB mechanism ( Supplementary Fig. S1 ), the structures of the key reaction intermediates are optimized and illustrated in Supplementary Fig. S4 , numbered from 6–12 sequentially. The overall potential energy graphs for all of the steps with the transition states are illustrated in Fig. 4b . The thermodynamic parameters of the elementary step ( Supplementary Table S2 ) indicate that the VB mechanisms can proceed with |e| U value of 2.56 eV in Steps V1~V3. For instance, Step V2 proceeds through the splitting of H 2 O on a Ti-5c site (7+h + →8+H + ) to produce an adsorbed OH that simultaneously leads to Ti-O rupture (State 8, Supplementary Figs S1 and S4 ). In the photocatalytic process, the Δ G value of the elementary step involving proton and hole should deduct the energy (|e| U ) of electron-hole pair generation. The U is the electropotential of a hole (at the maximum of the VB) with respect to standard hydrogen electrode ( U =0, Δ G H =0), and thus, |e| U represents the energy required to generate the electron-hole pair (a detailed description is given in Supplementary Note 2 ). However, Step V4 is the rate-controlling step in the VB mechanism. The |e| U value of 2.56 eV is not sufficiently large to overcome the high E a to drive the elementary reaction. In Step V4, the second H 2 O molecule attacks the O-O bond to form the structure of Ti-O-OH O-Ti (State 10), and proton removal with the photocatalytic evolution leaves oxygen radicals. Considering an overpotential of 1.22 V applied on the (001) surface, the Δ G of Step V4 can become negative because the |e| U equals 3.78 eV (2.56+1.22 eV). Furthermore, considering that the minimum CB of TiO 2 is higher in energy relative to standard hydrogen electrode by about 0.2 eV, the UV light above 3.98 eV (0.2+3.78 eV, ~310 nm) is sufficiently large to drive the photocatalytic NO formation reaction with H 2 O and h + on the VB of the TiO 2 (001) surface. The above mentioned protocols demonstrate that such a nitrate-producing process can be driven by the TiO 2 -mediated photocatalysis. Both thermodynamic and kinetic analyses reveal that the NO-forming process can spontaneously occur through the proposed CB mechanism, with a low E a in every step. However, the VB mechanism with a high E a needs overpotential to drive the photocatalytic reaction. As a consequence, the CB mechanism with a low E a can be the dominant pathway for the NO formation from quantum chemical calculations, and the VB mechanism can also possibly occur with h + at a low reaction rate. This is in agreement with the experimental results when both Cr(VI) dosing and ultrapure N 2 injection were applied. As the most important and widely used white paint component (~110 μg Ti mg −1 ) in the coating industry, the application of TiO 2 on the exterior walls of buildings and its consequent exposure to the atmosphere under UV light (for example, sunshine) irradiation is inevitable [10] , and in some cases extensive. Millions of tons of TiO 2 are produced per year and nearly 70% is used as a pigment in paints. Thus, the continual increasing production of nitrate on the surfaces of a large number of TiO 2 -coated buildings worldwide may be expected. Given the calculated nitrate-producing rate under ambient conditions ( Fig. 2c ), the increasing nitrate amount is estimated to be thousands of tons per day with the rough assumption that half of the pigment TiO 2 is exposed to the atmosphere under sunshine irradiation and 1 kg of TiO 2 can cover 5–10 m 2 of a building’s surface [15] . Considering the large amount of pigment TiO 2 used worldwide, the global production of nitrate per year from such processes, which is approximately equal to the NO x -N emission of biogenic substances from soils into the atmospheric environment in the United States of America in 2002 (ref. 16 ), could be impressive. Although these estimates are necessarily rough, this value suggests an undiscovered effect on the global nitrogen cycle as an abiotic process [17] , [18] . Owing to the universal personal use of TiO 2 to provide whiteness and opacity to products such as coatings, plastics, papers, inks, food and pills, an increasing number of toilets with TiO 2 coating inside, and buildings with TiO 2 coating outside in the form of glass coatings, cement, tiles and ceramics, the nitrate formation is expected to constantly increase [10] . The excess presence of nitrate in the environment is toxic to humans and aquatic lives. If the nitrate produced in TiO 2 -coated buildings is washed into water bodies, it can also contribute to water eutrophication and algae blooms, which are recognized as environmental disasters [18] . It should be noted that nano-sized TiO 2 particles (for example, <100 nm) are also widely used as a UV absorber in cosmetic and personal-care products, with a TiO 2 content ranging from 0.7 to 5.6 μg mg −1 (ref. 10 ). Our results imply that although TiO 2 particles are able to protect the skin from UV light, they may also produce nitrate simultaneously. At the present stage, it is unclear whether the nitrate formed on skin surfaces can penetrate the body, but it warrants further investigations. Reactions 1 and 2 suggest that NO can be produced in this process and released into the air. The NO formed from the TiO 2 -mediated photocatalysis would immediately react with O 2 and H 2 O to form NO 2 and nitrate [19] . NO is a prominent air pollutant that can lead to the formation of acid rains, photochemical smog or ozone and threaten human health [20] , [21] , [22] , [23] . In addition, when NO is exposed to oxygen, it can be converted into NO 2 , a brown toxic gas and air pollutant [24] . The unstable nitrous acid (HONO) [25] , [26] , which can be formed by NO 2 disproportionation on a range of surfaces including TiO 2 , fresh soot aerosol surfaces, glass, quartz and steel, can be rapidly decomposed into NO 2 , NO and H 2 O [27] , [28] , or be converted into NO and HO through photolytic decomposition [29] . Thus, HONO may also participate in the TiO 2 -mediated photocatalytic nitrate-producing process. It is worth noting that the nitrate-producing rate under outdoor conditions was higher than that in the indoor experiments ( Figs 1c , 2 ). This might be partially attributed to the presence of nitrogen oxides outdoors. The greatest nitrate-producing rate under ambient conditions was obtained in the morning (8:30–11:00) with the highest relative humidity and medium illumination intensity ( Fig. 2c ). This might be partially associated with the peak NO/NO x concentration in the morning rush hour in urban areas [26] , [30] . Such a rapid nitrate reduction can help decreasing the NO/NO x concentration in the air. Therefore, attention should be given to the worldwide use of TiO 2 and its potential environmental impacts. Such a direct TiO 2 -mediated nitrate-producing process under UV or sunlight irradiation may have potential industrial applications because of its gentle reaction conditions and the abundant and free raw materials, that is, atmospheric N 2 and O 2 . In the current well-known industrial nitrate-producing processes, for example, the Ostwald process [4] , [5] , NH 3 is used as the raw material and noble metal catalysts and high reaction temperatures are required to complete the nitrate-producing reaction. However, this TiO 2 -mediated photocatalytic process could be completed under sunshine at ambient temperature, and thus has application potential. Further investigation is warranted to increase both its nitrate-producing rate and yield for practical use. In summary, we have demonstrated that nitrate could be formed from abundant atmospheric N 2 and O 2 on TiO 2 surfaces under either UV or sunlight irradiation. NO is suggested as an intermediate product in this process and its formation mechanisms are elucidated by both experimental measurements and theoretical calculations. This might be the first report on nitrate production from air in relation to the globally increased use of TiO 2 (for example, P25 and E171) under ambient conditions. Such a catalytic reaction has a double-edged consequence: it has the potential to become an increasing pollution source, but it could also be used as an alternative cost-effective alternative to the Ostwald process for nitrate production. Setup and operation of photocatalytic reactors A quartz glass cylinder (6.5 cm in height and 6 cm in diameter) filled with 150-ml ultrapure water, except when 0.01 mM Cr 2 O 7 2− was added as an electron scavenger [14] , was used as the photoreactor for photocatalytic reaction. The commercial TiO 2 nanoparticles, P25 (Degussa Co., Germany), and the widely used food-grade TiO 2 , E171 (<250 nm, Jianghutaibai Co., China), were, respectively, painted on a chemically stable carbon paper (GEFC Co., China) [31] and were inserted into the photoreactor for tests. A 30-W low-pressure mercury lamp was used as the source of UV light. The lamp was fixed outside the reactor against the TiO 2 -carbon paper surface at a 10 cm distance, with an intensity of 4.81±0.51 μW cm −2 at 253.7 nm. Air was purged into the reactor constantly and slowly through a flask, half of which was filled with ultrapure water for cooling and purification. In the control experiment, a mixture of ultrapure N 2 (99.999%) and ultrapure O 2 (99.995%) (3:1/v:v) was purged into the reactor 1 h before UV irradiation and lasted 72 more hours under UV irradiation. Blank experiments were also carried out with the injection of either purified air or ultrapure N 2 gas but in the absence of either UV irradiation or TiO 2 photocatalyst (with or without the carbon paper inserted into the photoreactor), or with the injection of ultrapure Ar gas or ultrapure N 2 gas and in the presence of UV irradiation. The solutions in the reactor were stirred constantly. The morphology of the prepared TiO 2 -carbon paper was imaged using SEM (FEI Co., the Netherlands) and its crystal structure was characterized using X-ray diffraction (X’ Pert PRO, Philips Co., the Netherlands). The effect of relative humidity on this photocatalytic process was evaluated in a climatic chamber under a constant temperature (25±0.1 °C) but with different set humidities. Outdoor experiments under solar light irradiation were also carried out. Ultrapure water was dropped on the TiO 2 -carbon paper surface at a rate of 3 ml h −1 to eliminate the interference of relative humidity and was collected. Then, ultrapure water was used to wash the TiO 2 -carbon paper and the beaker several times, and the water samples were collected into a 25-ml volumetric flask for measurement every 2.5 h. A luminometer (ZDS-10, Xuelian Co., China) was used to measure the illuminance intensity on the TiO 2 -carbon paper surface every 0.5 h. Experiments using the TiO 2 (P25 or E171) on carbon paper under solar light irradiation but in the absence of ultrapure water were also conducted for comparison. Analysis of intermediates and final products To identify the possible intermediate products formed in this process, a separate photocatalytic experiment was carried out in a 250-ml airtight glass reactor, in which 150-ml ultrapure water and 0.1-g TiO 2 (P25) powders were added. The reactor was equipped with a quartz glass window (2 × 4 cm 2 ) and a sample outlet capped using a rubber stopper. The liquid samples were taken from the sample outlet of the reactor by using an injector and were used for analysis. There was a gas circuit between this reactor and a 5-l flask filled with air. A peristaltic pump was used to ensure sufficient airflow through the reactor during the 3-day reaction process. The gas samples in the airtight reactor before and after the 3-day photocatalytic reaction were analysed with a gas chromatograph (6890, Agilent Co., USA) equipped with an electroncapture detector, and a FTIR (TENSOR 27, Bruker Co., Germany) equipped with a mercury-cadmium-teluride detector for qualitative and quantitative analyses of the potential NO x intermediates. Both nitrate and nitrite were analysed using an ion chromatograph (ICS-1000, Dionex Co., USA) and ammonia was determined using a spectrophotometer (UV2540, Shimdzu HIMADZU, Japan) at a wavelength of 420 nm after the Nessler reaction. All of the organic and inorganic reagents used were of analytical grade, unless otherwise stated. All of the solutions were prepared with ultrapure water (Millipore Co., USA). All of the tests were conducted in triplicate. Quantum chemical calculations The formation mechanisms of intermediate gaseous products on the (001) surface of the nanoscale TiO 2 was explored with first-principles density functional theory calculations (details are provided in Supplementary Methods ). The (001) facet, which is the minor surface in the equilibrium shape of the anatase nanocrystals in TiO 2 P25 (Degussa), is found to be the dominant active site and contributes to the unique properties of TiO 2 nanoparticles in the form of anatase. Its existence in anatase TiO 2 has been demonstrated theoretically and experimentally [32] , [33] , [34] . The structures of the reactants, intermediates and products in the reaction process at the (001) surface of nanoscale TiO 2 were optimized in water solvation. The potential energy profiles and the Gibbs free energy changes of each step for the intermediate formation were calculated. Geometry parameters of O-O and N-N in the intermediate states of pathways were calculated. Finally, the reaction mechanisms for the intermediate product formation were elucidated. How to cite this article: Yuan, S.-J. et al. Nitrate formation from atmospheric nitrogen and oxygen photocatalysed by nano-sized titanium dioxide. Nat. Commun. 4:2249 doi: 10.1038/ncomms3249 (2013).